Microbial interactions shape cheese flavour formation Cheese fermentation and flavour formation are the result of complex biochemical reactions driven by the activity of multiple microorganisms. Here, we studied the roles of microbial interactions in flavour formation in a year-long Cheddar cheese making process, using a commercial starter culture containing Streptococcus thermophilus and Lactococcus strains. By using an experimental strategy whereby certain strains were left out from the starter culture, we show that S. thermophilus has a crucial role in boosting Lactococcus growth and shaping flavour compound profile. Controlled milk fermentations with systematic exclusion of single Lactococcus strains, combined with genomics, genome-scale metabolic modelling, and metatranscriptomics, indicated that S. thermophilus proteolytic activity relieves nitrogen limitation for Lactococcus and boosts de novo nucleotide biosynthesis. While S. thermophilus had large contribution to the flavour profile, Lactococcus cremoris also played a role by limiting diacetyl and acetoin formation, which otherwise results in an off-flavour when in excess. This off-flavour control could be attributed to the metabolic re-routing of citrate by L. cremoris from diacetyl and acetoin towards α -ketoglutarate. Further, closely related Lactococcus lactis strains exhibited different interaction patterns with S. thermophilus , highlighting the significance of strain specificity in cheese making. Our results highlight the crucial roles of competitive and cooperative microbial interactions in shaping cheese flavour profile. Fermented foods based on microbial consortia (e.g., cheese, kefir and kombucha) constitute a large part of the modern diet with many reported health benefits [1] , [2] , [3] . In cheese, well defined Starter Lactic Acid Bacteria (SLAB) cultures are used to ensure consistent and flavourful products. During cheese making, microbes encounter dynamic conditions characterized by different nutrient availability and different stresses, starting with an initial feast during milk fermentation, followed by a long period of famine during cheese ripening. Cheese-making thus provides a controlled system with well characterized dynamics to understand the role of microbial interactions in shaping the characteristics and quality of fermented foods [4] . In industrial cheese making, SLAB cultures are responsible for milk acidification via lactose fermentation. They are predominantly composed of mesophilic strains of Lactococcus , including the species L. lactis and L. cremoris as well as thermophilic strains of Streptococcus thermophilus . A rich literature exists on the physiology of the species in mono-cultures [5] , [6] , [7] , [8] , and genome-scale metabolic models have been used to model their metabolism [9] , [10] , [11] . In contrast, the interactions between the three taxa is still largely unknown from a mechanistic perspective despite indications of strong inter-dependencies [12] , [13] . Further, the current knowledge on cheese microbial interactions is limited to the scope of simplified artificial milk media, concerns pairwise associations, or focus only on the short time interval during the milk acidification. Less is known about the interactions involving more than two SLAB strains and how interaction networks evolve during the cheese ripening steps. Metabarcoding and metagenomics approaches have also been used to study the cheese microbiome [14] , [15] , [16] . While these studies provide a good overview on the community dynamics during cheese-making using higher-order taxonomy, they are limited in uncovering inter-species interactions and strain-level diversity. In this study, we investigated the role of microbial interactions and interacting agents in cheese flavour formation. We employed a strain dropout strategy, which involves omitting either a single strain or a group of strains from the starter culture. Subsequently, we conducted a comprehensive characterization of the entire cheese-making process. We used an industrially relevant SLAB culture, containing: one Streptococcus thermophilus (ST), two major L. lactis (LLm1 & LLm2), one major L. cremoris (LC), and a mixture of 21 L. cremoris and L. lactis strains in smaller fractions (hereafter, Lactococcus blend (LB)). We investigated the effect of leaving out S. thermophilus and Lactococcus blend in a year-long Cheddar-making experiment (Fig. 1 a). Subsequently, controlled milk experiments were conducted to delve into the potential role of interactions, aiming to elucidate the observed growth advantage of Lactococcus from S. thermophilus . For the latter, we used an integrative systems biology approach that combined multiple layers of biological information from genomics, genome-scale metabolic modeling, metatranscriptomics to metabolomics (Fig. 1 b). Fig. 1: Schematic representation of the experimental design and methods. a The 1 year long cheddar-making experiment. The SLAB culture is composed of one S. thermophilus (ST), two major L. lactis strains (LLm1 & LLm2), one major L. cremoris (LC), and a blend of Lactococcus strains (LB). Microbial population dynamics were quantified during cheese ripening using a selective method of viable cell counting, which discriminates between thermophilic cocci, mesophilic cocci and non-Starter Lactic Acid Bacteria (non-SLAB). Additionally, metabolic changes in the cheeses were measured using several targeted analytical chemistry approaches measuring acids, sugars, flavour-related organic compounds and peptides. b Schematic representation of the controlled milk experiment in the laboratory as well as of the methods (1–5) used in the controlled milk experiment. This second experiment involves the removal of additional strains, namely the individual exclusion of three major Lactococcus strains. The numbers indicate the different types of data and analysis as follows: 1. metatranscriptomics, 2. metabolomics (i.e., acids, sugars, flavour-related organic compounds), 3. genomics, 4. phylogenomics and 5. genomes-scale metabolic models (GEMs) and community simulations. Our integrative systems biology approach combined: (i) the analysis of the SLAB community’s genomes, (ii) the generation and simulation of their respective GEMs, (iii) the analysis of the metatranscriptomes across the different strain removal conditions and (iv) the quantification of key metabolites. Full size image S. thermophilus supports the growth of lactoccoci and shapes the metabolite profile during cheese ripening To study the interactions between the members of the SLAB culture, we started by quantifying the population dynamics during a year-long ripening cheese making experiment (see Methods). We used four variations of starter cultures: (i) containing all member species of an industrial starter culture, viz ., S. thermophilus (ST), L. cremoris (LC), L. lactis (LLm1 and LLm2), and Lactococcus blend (LB); (ii) the same as (i) but prepared independently (HP); (iii) excluding LB; and (iv) excluding ST (Fig. 1 a). In the three conditions that included S. thermophilus , we observed a trend of slow decline in the population of lactoccoci and S. thermophilus , starting with 9.25 and ending at 8 log10 CFU/g (Fig. 2 a–c). In the single condition that excluded S. thermophilus , we observed a much steeper decline in lactoccoci population, ending at 6.5 log10 CFU/g (Fig. 2 a, b). Also, the declining lactoccoci population exhibited different trajectories between the two batches, albeit both converging at 9 and 12 months (Fig. 2 a, b). The non-SLAB count increased from 0 to 7.5 log10 CFU/g, in the highest case (Fig. 2 d). Based on 95% confidence interval estimates, we observed high variability among the non-SLAB populations, but with no appreciable overall difference between the conditions (Fig. 2 d). Leaving out Lactococcus blend or changing the way of packing the different strains in the culture did not result in any visible response to the community dynamics. Thus, inter-species interactions, especially involving S. thermophilus , appear to be driving the overall population dynamics. Fig. 2: S. thermophilus benefit the growth of lactoccoci community and influence the final flavour of cheese. a–d Microbial population dynamics during cheese ripening. Relationship between CFUs and time (months) for ( a ) Mesophilic, ( c ) Thermophilic cocci, and ( d ) non-Starter Lactic Acid Bacteria (non-SLAB). The mean values are represented by lines, symbols (circle and asterisk) indicate batch experiments, and the shaded area reflect the 95% confidence interval estimates (similarly in h ). b Presents the boxplot comparison of the different condition on Mesophilic cocci at 12 months. The box edges represent the interquartile range, the ends of the whiskers represent ± 1.5 × the interquartile range and central lines are the median values (similarly in f ). The p -values of two-sided t test presented as ns: p > 0.05, * p < = 0.05, **** p < = 0.0001. Note, significant reduction only on Mesophilic cocci is observed when S. thermophilus is absent. Condition All corresponds to whole culture which is composed of 25 number of strains. HP corresponds to an alternative method (hand packed) of the whole culture inoculation. -LB corresponds to the removal of a L. lactis blend population. -ST corresponds to the removal of the S. thermophilus strain. e–h Metabolome dynamics during cheese ripening. e 2-dimensional representation with the usage of UMAP of all samples based on the metabolomics measurements (acids, carbohydrates and peptides). The colour indicates the time when the sample was taken and the shape indicates the four different conditions. Note, the stronger change is observed between 2 week and 3 months while the removal of ST (cross symbol) has a strong effect on the later time of cheese ripening. f Relative change of the metabolites on different time intervals including all the conditions, both colour and shape indicates the class of the metabolite. Note, the higher relative change of peptides followed by acids at the interval between 2 week and 3 months, later acids exhibit higher changes. The three measured sugars (glucose, lactose and galactose) are excluded from this panel. g Selection of the six most discriminative metabolites out of 50 for the four conditions. Colour indicate the condition while the right side shape the class of the metabolite. Note, the majority of peptide concentrations are significant different when S. thermophilus is not present, as well as with galactose, lactose and lactic acid. The amino acid sequences of the peptides presented ( g ) in top-down order are EEEKNRLNF, VNELSKD and ELSKDIGSESTE. h Galactose concentration over time highlights the absence of galactose when S. thermophilus is absent. The galactose concentration remains steady from the start till the 9 month of cheese ripening and then shows signs of decline. All panels are based on n = 4 biologically independent samples. Full size image To measure the effect of the microbial interactions in the resulting phenotype of the cheese, we used targeted metabolomics analyses. Across conditions, the biggest change in the metabolic profiles of cheese was observed between the two-week mark and three months (Fig. 2 e). This can be attributed to changes in peptide composition followed by the general increase in amino acids concentrations (Fig. 2 f). Furthermore, cheese metabolomes continue to change at a slower pace between the three- to twelve-month marks, resulting in different end profiles. A notable time-depended accumulation of compounds after the third month was observed on acetic acid, tyramine, g-amino butyric acid, putrescine and cadaverine (Fig. 2 f and Supplementary Fig. 1) . The cheeses produced without S. thermophilus formed a separate cluster relative to the rest (Fig. 2 e). This pattern can be ascribed to compounds that, over time, result in significantly different concentrations across strain removal conditions, especially when S. thermophilus was absent. The majority of these compounds are peptides that were either not accumulated, accumulated in lower amounts or accumulated in higher amounts without the addition of S. thermophilus (Supplementary Fig. 2) . Lactose, galactose and lactic acid concentrations were also found to be significantly different when S. thermophilus was absent (Fig. 2 g, ANOVA F (3,36) = 208 ± 334, p < 0.001, η 2 = 0.86 ± 0.08). Specifically, lactose was not fully consumed and galactose was not produced when S. thermophilus was absent (Supplementary Fig. 3 c). This difference was already notable in the samples from the second week of cheese ripening and remained relatively constant until the end of cheese-making (Fig. 2 h and Supplementary Fig. 3 a, c and e). These results point towards the significant influence of S. thermophilus growth during milk fermentation, while the over-time differentiation, for example on peptide composition, indicates the important effect of non-growing yet active cells during long-term cheese ripening. The presence of S. thermophilus was found to benefit both the growth of the Lactococcus community and the final metabolic profile of the cheddar cheese. Notably, the growth benefit is not clearly visible before two weeks to three months, a time-frame that may be considered prohibitively long for experiments in the laboratory. Instead, these effects become more evident as the experimental time-frame expands to one year. The observed effect may be attributed to the early S. thermophilus overflow metabolites during milk fermentation or to alteration of its metabolism at near-zero growth rates during cheese ripening [7] , [17] , [18] . In both cases leading to potentially promoting cross-feeding interactions [6] . It cannot be ruled out that the release of distinct cytoplasmic enzymes through the lysis of S. thermophilus could enhance the growth of Lactococcus [19] , [20] . Consequently, these factors could result in the identified differences in peptide composition in the final cheese. In accordance with the literature, the presence of S. thermophilus reveals a few key metabolic changes from the milk fermentation; the complete consumption of lactose and the production of galactose [17] , [18] . Together, the compositional and metabolic profiles led us to conclude that both early and late S. thermophilus activity is critical for the long term effect on Lactococcus population and cheese flavour development. S. thermophilus has strain-specific interactions with the members of Lactococcus lactis community To assess the role of S. thermophilus , we performed controlled experiments wherein additional strains were removed (Fig. 1 b). Samples were taken when milk fermentation reached the transition from exponential to stationary phase (at pH 5) and gene expression was monitored using metatranscriptomics. To further investigate the microbial interactions within the SLAB culture, we also analyzed the genomes of the individual strains in the culture and their phylogenetic relationship (Fig. 3 a). The phylogenomic analysis separated the species L. lactis and L. cremoris into two distinct groups. Two of the main Lactococcus strains, LC and LLm2, have no close relatives within the culture community. For the third main Lactococcus strain, LLm1, we identified two close relatives (LL-LB01 and LL-LB02), belonging to the Lactococcus blend (Fig. 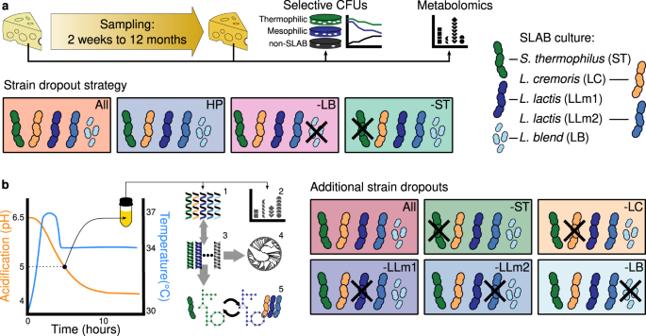Fig. 1: Schematic representation of the experimental design and methods. aThe 1 year long cheddar-making experiment. The SLAB culture is composed of oneS. thermophilus(ST), two majorL. lactisstrains (LLm1 & LLm2), one majorL. cremoris(LC), and a blend ofLactococcusstrains (LB). Microbial population dynamics were quantified during cheese ripening using a selective method of viable cell counting, which discriminates between thermophilic cocci, mesophilic cocci and non-Starter Lactic Acid Bacteria (non-SLAB). Additionally, metabolic changes in the cheeses were measured using several targeted analytical chemistry approaches measuring acids, sugars, flavour-related organic compounds and peptides.bSchematic representation of the controlled milk experiment in the laboratory as well as of the methods (1–5) used in the controlled milk experiment. This second experiment involves the removal of additional strains, namely the individual exclusion of three majorLactococcusstrains. The numbers indicate the different types of data and analysis as follows: 1. metatranscriptomics, 2. metabolomics (i.e., acids, sugars, flavour-related organic compounds), 3. genomics, 4. phylogenomics and 5. genomes-scale metabolic models (GEMs) and community simulations. Our integrative systems biology approach combined: (i) the analysis of the SLAB community’s genomes, (ii) the generation and simulation of their respective GEMs, (iii) the analysis of the metatranscriptomes across the different strain removal conditions and (iv) the quantification of key metabolites. 3 and Supplementary Table 1) . The rest of the strains in the Lactococcus blend formed distinct sub-clusters within the cremoris clade (Fig. 3 ). By employing pan-genome analysis on Lactococcus strains, we identified singletons (i.e., a gene found only in one genome) for each member of the culture. The highest number of singletons was harbored by the main LLm2 followed by LC, and LLm1 where its number of singletons was in the same range as the Lactococcus blend strains, with numbers 288, 134, 79 and average of 53.6 ± 18.6, respectively (Fig. 3a ). In parallel, we evaluated both the presence and activity level (using metatranscriptomics) of the Lactococcus strains by calculating percentile of the transcribed singletons per genome. We found a high number of transcribed singletons on all the main Lactococcus strains, while this number varied considerably among the strains of the Lactococcus blend, raising questions regarding whether or not these strains were active (Fig. 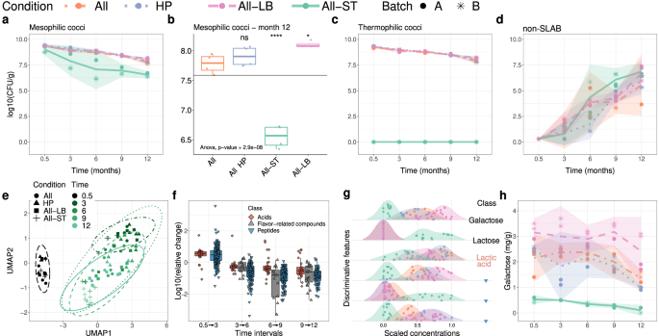Fig. 2:S. thermophilusbenefit the growth of lactoccoci community and influence the final flavour of cheese. a–dMicrobial population dynamics during cheese ripening. Relationship between CFUs and time (months) for (a) Mesophilic, (c) Thermophilic cocci, and (d) non-Starter Lactic Acid Bacteria (non-SLAB). The mean values are represented by lines, symbols (circle and asterisk) indicate batch experiments, and the shaded area reflect the 95% confidence interval estimates (similarly inh).bPresents the boxplot comparison of the different condition on Mesophilic cocci at 12 months. The box edges represent the interquartile range, the ends of the whiskers represent ± 1.5 × the interquartile range and central lines are the median values (similarly inf). Thep-values of two-sidedttest presented as ns:p> 0.05, *p< = 0.05, ****p< = 0.0001. Note, significant reduction only on Mesophilic cocci is observed whenS. thermophilusis absent. Condition All corresponds to whole culture which is composed of 25 number of strains. HP corresponds to an alternative method (hand packed) of the whole culture inoculation. -LB corresponds to the removal of aL. lactisblend population. -ST corresponds to the removal of theS. thermophilusstrain.e–hMetabolome dynamics during cheese ripening.e2-dimensional representation with the usage of UMAP of all samples based on the metabolomics measurements (acids, carbohydrates and peptides). The colour indicates the time when the sample was taken and the shape indicates the four different conditions. Note, the stronger change is observed between 2 week and 3 months while the removal of ST (cross symbol) has a strong effect on the later time of cheese ripening.fRelative change of the metabolites on different time intervals including all the conditions, both colour and shape indicates the class of the metabolite. Note, the higher relative change of peptides followed by acids at the interval between 2 week and 3 months, later acids exhibit higher changes. The three measured sugars (glucose, lactose and galactose) are excluded from this panel.gSelection of the six most discriminative metabolites out of 50 for the four conditions. Colour indicate the condition while the right side shape the class of the metabolite. Note, the majority of peptide concentrations are significant different whenS. thermophilusis not present, as well as with galactose, lactose and lactic acid. The amino acid sequences of the peptides presented (g) in top-down order are EEEKNRLNF, VNELSKD and ELSKDIGSESTE.hGalactose concentration over time highlights the absence of galactose whenS. thermophilusis absent. The galactose concentration remains steady from the start till the 9 month of cheese ripening and then shows signs of decline. All panels are based onn= 4 biologically independent samples. 3 a and Supplementary Table 2 ). We hypothesized that the temperature dynamics during the experiment could influence the strain acidification potential. To test this, by carrying out milk fermentation using each of the individual Lactococcus strains at different temperatures, we calculated a proxy for their temperature stress tolerance (Pearson correlation between curves of 30 °C against 37 °C, 40 °C and 43 °C). The results showed that the L. lactis strains have higher temperature stress tolerance in the tested ranges, including Lactococcus blend strains LL-LB01 and LL-LB02 (PCC 0.96 ± 0.05). The L. cremoris strains exhibited low temperature stress tolerance (PCC 0.7 ± 0.24), with the main LC being one of the most stress tolerant strains within this group (PCC range 0.84–0.99) (Fig. 3a and Supplementary Fig. 4 a, b). Fig. 3: The removal of different Lactococcus strains has a distinct effect on gene expression in S. thermophilus . a–e relationship of the Lactococcus phylogeny with the S. thermophilus transcription change on different dropout conditions. a Lactococcus phylogenetic tree separates the L. cremoris and L. lactis strains. The two clades are coloured with transparent yellow and gray, respectively. The colours and shape of the tree tips indicate the strains presents in the SLAB culture. Orange triangles represent L. cremoris (LC), dark and light blue circles represent L. lactis (LLm1 and LLm2), and a teal square represents the Lactococcus blend (LB). Tree empty tips correspond to the obtained complete NCBI genomes of Lactococcus . Additional information is presented in the outer layers of the tree. The first layer presents the unique k-mer content based on the SLAB culture’s genomes (purple-scale colour) and indicates higher number for the strains who have no close relative within the culture. The second layer presents the proxy of temperature stress tolerance based on Pearson Correlation Coefficient (PCC) between individual acidification curve of 30 °C and 40 °C (red-scale colour). High values correspond to high temperature tolerance. The clade L. cremoris shows lower temperature tolerance, with few exceptions including the main LC strain (more details presented in Supplementary Fig. 5 ). The third layer presents the percentile of transcribed sigletons (green-scale colour) as well as the total number of the strains sigletons (outer bars). b–e Volcano plots show the S. thermophilus transcription between the whole community (All) and the different Lactococcus dropout conditions, respectively. The colours correspond to the 4 Lactococcus components. The S. thermophilus transcription was observed to change more when LLm1 was left out followed by LB, with 291 and 182 number of total significant up/down regulated genes, respectively. A smaller effect of 21 genes was observed when LC was left out and only one gene when LLm2 was left out. Full size image We next explored the extent to which we could discriminate between the different strains. The number of unique k-mers in each genome ranged from 368 to 622,455 and they were found to be dependent on the presence of close phylogenetic relative strains (Fig. 3 a). The k-mer transcription abundance indicated the feasibility of discriminating between the three main Lactococcus strains (LC, LLm1 and LLm2) and the one S. thermophilus strain, but not between the strains in the Lactococcus blend (Supplementary Fig. 5 ). Using differential expression analysis, we investigated the interaction effect on S. thermophilus transcriptome by leaving out each Lactococcus strain/blend from the culture. We found the strongest response when LLm1 was left out followed by Lactococcus blend, LC and LLm2 with 291, 182, 21 and 1 gene(s) significantly differential expressed, respectively (Fig. 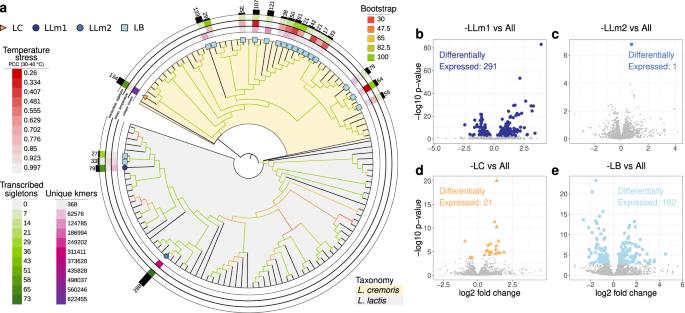Fig. 3: The removal of differentLactococcusstrains has a distinct effect on gene expression inS. thermophilus. a–erelationship of theLactococcusphylogeny with theS. thermophilustranscription change on different dropout conditions.aLactococcusphylogenetic tree separates theL. cremorisandL. lactisstrains. The two clades are coloured with transparent yellow and gray, respectively. The colours and shape of the tree tips indicate the strains presents in the SLAB culture. Orange triangles representL. cremoris(LC), dark and light blue circles representL. lactis(LLm1 and LLm2), and a teal square represents the Lactococcus blend (LB). Tree empty tips correspond to the obtained complete NCBI genomes ofLactococcus. Additional information is presented in the outer layers of the tree. The first layer presents the unique k-mer content based on the SLAB culture’s genomes (purple-scale colour) and indicates higher number for the strains who have no close relative within the culture. The second layer presents the proxy of temperature stress tolerance based on Pearson Correlation Coefficient (PCC) between individual acidification curve of 30 °C and 40 °C (red-scale colour). High values correspond to high temperature tolerance. The cladeL. cremorisshows lower temperature tolerance, with few exceptions including the main LC strain (more details presented in Supplementary Fig.5). The third layer presents the percentile of transcribed sigletons (green-scale colour) as well as the total number of the strains sigletons (outer bars).b–eVolcano plots show theS. thermophilustranscription between the whole community (All) and the differentLactococcusdropout conditions, respectively. The colours correspond to the 4Lactococcuscomponents. TheS. thermophilustranscription was observed to change more when LLm1 was left out followed by LB, with 291 and 182 number of total significant up/down regulated genes, respectively. A smaller effect of 21 genes was observed when LC was left out and only one gene when LLm2 was left out. 3 b–e, Supplementary Table 3 and sections below). Although both LLm1 and LLm2 belong to L. lactis clade, the latter strain stands out by having the highest number of singletons as well as having the second highest number of unique k-mers (Fig. 3 ). By removing strains with a different degree of relatedness we identified that different Lactococcus strains have distinct effects on gene expression of S. thermophilus . This finding can be attributed to the different genetic background and the diverse phylogenetic relationships within the Lactococcus community [21] , highlighting the diversity of potential microbial interactions between S. thermophilus and the Lactococcus community. S. thermophilus proteolytic activity may benefit Lactococcus community by providing nitrogen sources To investigate mechanisms of inter-species interactions, we generated genome-scale metabolic models for the individual strains in the culture and performed flux balance analysis-based simulations. To explore the effect of changes in growth medium composition, we generated models gap-filled on relevant variations of milk-mimicking media. Supplementary Fig. 6 a shows overall model statistics for the different species, while Supplementary Fig. 6 b shows the specific reactions added through gap-filling on different media across the models (see Supplementary Note 1 ). Flux balance simulations with individual models were carried out using the different model sets in aerobic and anaerobic variants of fermented and non-fermented milk (Fig. 4 a, b and Supplementary Fig. 6 c, d). All species consistently consumed lactose in simulations where growth was feasible. Several differences in amino acid uptake/secretion were observed among the strains. The branched chain amino acid valine was exported by S. thermophilus in all but one simulation condition, whereas LC, LLm1, and LLm2 consumed this amino acid in four, six, and three simulations conditions, respectively. Additional amino acid uptake/secretion predictions are reported at Supplementary Note 1 . Fig. 4: S. thermophilus provides nitrogen in form of amino acids to L. lactis community, which is necessary for de novo nucleotide biosynthesis. a Summary of metabolic modeling analysis including individual model and community-based simulations. b Selected exchange fluxes predicted across individual flux balance analysis simulations carried in milk media variations for each set of metabolic models. In particular fermentation products, amino acids, and carbon sources highlighting differences in metabolic strategies across species. c Alluvial diagram showing predicted metabolic exchanges from community simulations in milk media variants, highlighting the fact the amino acid valine is strongly predicted across all simulation conditions where metabolic cross-talk is expected. The four metabolic models used correspond to L. cremoris (LC), coloured orange; L. lactis (LLm1 and LLm2), coloured dark and light blue; and S. thermophilus (ST), coloured green. Refer to Supplementary Fig. 6 for more details on the metabolic models and simulation. d–i Transcriptomic profiles between All and -ST ( S. thermophilus is left out) conditions of key functions for all the strains in SLAB culture. The box edges represent the interquartile range, the ends of the whiskers represent ± 1.5 × the interquartile range and central lines are the median values ( n = 3 biologically independent samples). d–f Transcriptomics boxplots of branched chain amino acids (BCAA) aminotransferase, BCAA transport system 2 carrier protein and ammonium transporter (T) supports the predictions of metabolic exchanges. Note, ( e ) the higher transcription profile of S. thermophilus on BCAA transport system. g–j Up-regulation of Lactococcus glutamine and nucleotide metabolism when S. thermophilus is left out. g–i Boxplots present the activities of nitrogen regulatory protein P-II, glutamine synthetase (glnA) and related transcriptional regulator (TR) (GlnR) for all community members. Note, the up-regulation of all the enzymes derived from Lactococcus strains when S. thermophilus is left out. j Metatranscriptomics represents the increased activity of Lactococcus reactions, which are incorporated into Escher maps. The pattern shows a coordinate up-regulation (with green) of the enzymes towards guanine biosynthesis (and uridine). k Schematic compilation of the compounds S. thermophilus may provide to Lactococcus community as well as selected transcriptional changes of the Lactococcus community when S. thermophilus was left out. The colour and direction of the arrows represent the up- and down- regulation with green/up and red/down, respectively. Full size image To assess potential cross-feeding, we performed community simulations using the SMETANA framework (see Supplementary Note 1 ). We used the calculated SMETANA scores, ranging from 0 to 1, as a measure of predicted interaction confidence (0 being lowest confidence and 1 being the highest) [22] . These simulation indicate that S. thermophilus provides valine to Lactococcus strains in all three community simulation conditions (gap-filled on rich aerobic milk & simulated on minimal aerobic milk, gap-filled on rich anaerobic milk & simulated on minimal aerobic milk, and gap-filled on rich anaerobic milk & simulated on minimal anaerobic milk) where exchanges were predicted between community members (Fig. 4 c). Not only was this interaction consistent, it also occurred with a SMETANA score of 1 in every case, suggesting that this is a key ecological interaction for maintaining the composition and function of the community. Serine exchanges from S. thermophilus to LLm1 were predicted in 2 out of 3 community simulation conditions, with an average SMETANA score of 0.38 ± 0.01. Exchanges from S. thermophilus to LC involving glycine and ammonium were predicted in 1 out of the 3 simulation conditions, with SMETANA scores of 0.3 and 0.29, respectively (Fig. 4 c). Finally, an exchange from S. thermophilus to LLm2 involving alanine was predicted under only 1 simulation condition with a SMETANA score of 0.42. Overall, the metabolic simulations strongly indicate cross-feeding between the community members, with S. thermophilus standing out as a key donor (Fig. 4 c). To complement the genomic and metabolic modeling analysis, we investigated the changes in S. thermophilus and Lactococcus community transcriptome. The principal component analysis (Supplementary Fig. 7 ) showed pattern consistency with the differential transcriptome analysis (Fig. 3 b–e, Supplementary Note 2 ). Regarding changes in S. thermophilus ’s transcriptome, we found up-regulated genes annotated as oligopeptide-binding protein (AmiA) and oligopeptide transport system permease protein (OppB, OppC, OppD & OppF) (see Supplementary Note 2 ). Seven down-regulated genes are annotated as transporters, such as glutamine ABC transporter permease protein (GlnP), cadmium, cobalt and zinc/H(+)-K(+) antiporter (Supplementary Note 2 ). Further, transcriptional repressors such as the catabolite control protein A (CcpA) and nitrogen-metabolism-regulating-proteins such as GTP-sensing transcriptional pleiotropic repressor (CodY) were found to be transcriptionally active. In line with the putative interactions predicted using metabolic modeling, we found a gene annotated as branched-chain amino acids (BCAA) transaminase expressed in S. thermophilus , suggesting that valine biosynthesis is active. Moreover, we found a gene annotated as BCAA transport system 2 carrier protein (BrnQ) as well expressed, suggesting that S. thermophilus is secreting valine. Complementary differential pathway enrichment analysis supported further that valine biosynthesis was enriched in S. thermophilus metatranscriptome (Fig. 4 d, e). Overall, the metabolic modeling and metatranscriptome analysis together suggests that S. thermophilus can act as a branched chain amino acid donor to Lactococcus . It is well known that Lactococcus harbor a number of amino acid auxotrophies including valine [1] , [20] , [23] , [24] . In addition, the SMETANA simulations provide insights into the metabolic strategies that may be employed by community members under challenging media conditions. We next investigated transcriptional change in the Lactococcus community in the presence and absence of S. thermophilus . As it is not possible to distinguish between the transcriptome profiles of all the different Lactococcus strains, we merged these into one group for pan-genome analysis and pan-metabolic modeling. Strain-to-strain transcriptional changes were investigated when possible (see Supplementary Note 2 ). The most up-regulated OGs in Lactococcus when S. thermophilus is left out are involved in nitrogen assimilation, namely nitrogen regulatory protein P-II, related transcriptional regulator (GlnR), ammonium transporter (amtB), glutamine synthetase (glnA) and glutamine transport ATP-binding protein (glnQ). Additionally, we confirmed that GlnR in Lactococcus regulates the three operons, namely amtB, glnA, and glnQ (Fig. 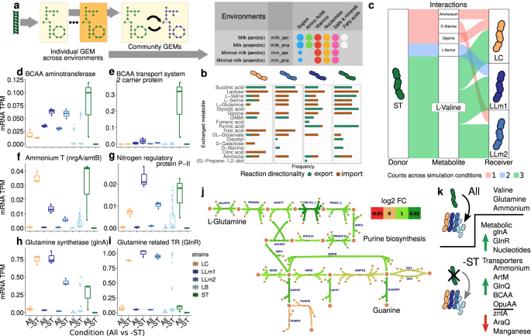Fig. 4:S. thermophilusprovides nitrogen in form of amino acids toL. lactiscommunity, which is necessary for de novo nucleotide biosynthesis. aSummary of metabolic modeling analysis including individual model and community-based simulations.bSelected exchange fluxes predicted across individual flux balance analysis simulations carried in milk media variations for each set of metabolic models. In particular fermentation products, amino acids, and carbon sources highlighting differences in metabolic strategies across species.cAlluvial diagram showing predicted metabolic exchanges from community simulations in milk media variants, highlighting the fact the amino acid valine is strongly predicted across all simulation conditions where metabolic cross-talk is expected. The four metabolic models used correspond toL. cremoris(LC), coloured orange;L. lactis(LLm1 and LLm2), coloured dark and light blue; andS. thermophilus(ST), coloured green. Refer to Supplementary Fig.6for more details on the metabolic models and simulation.d–iTranscriptomic profiles between All and -ST (S. thermophilusis left out) conditions of key functions for all the strains in SLAB culture. The box edges represent the interquartile range, the ends of the whiskers represent ± 1.5 × the interquartile range and central lines are the median values (n= 3 biologically independent samples).d–fTranscriptomics boxplots of branched chain amino acids (BCAA) aminotransferase, BCAA transport system 2 carrier protein and ammonium transporter (T) supports the predictions of metabolic exchanges. Note, (e) the higher transcription profile ofS. thermophiluson BCAA transport system.g–jUp-regulation ofLactococcusglutamine and nucleotide metabolism whenS. thermophilusis left out.g–iBoxplots present the activities of nitrogen regulatory protein P-II, glutamine synthetase (glnA) and related transcriptional regulator (TR) (GlnR) for all community members. Note, the up-regulation of all the enzymes derived fromLactococcusstrains whenS. thermophilusis left out.jMetatranscriptomics represents the increased activity ofLactococcusreactions, which are incorporated into Escher maps. The pattern shows a coordinate up-regulation (with green) of the enzymes towards guanine biosynthesis (and uridine).kSchematic compilation of the compoundsS. thermophilusmay provide toLactococcuscommunity as well as selected transcriptional changes of theLactococcuscommunity whenS. thermophiluswas left out. The colour and direction of the arrows represent the up- and down- regulation with green/up and red/down, respectively. 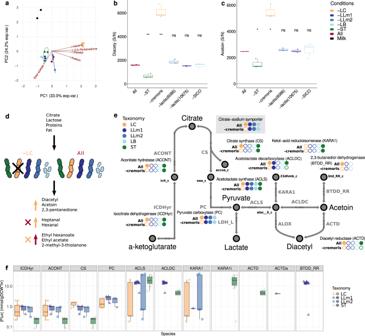Fig. 5: Cheese flavour compounds are strongly influenced by the interactions withinLactococcuscommunity. The measured metabolome from the controlled milk experiments in response to strain removal conditions (a–d).aThe PCA of key carbohydrades, acids and cheese flavour compounds. The strongest response was observed from the removal ofL. cremoris, followed by a coordinated response of LLm1, LB andS. thermophilus. Removal of LLm2 does not affect the measured metabolome. The arrows represent the top 5 compounds responsible for the observed changes (2,3-pentanedione, hexanal, diacetyl, acetoin and ethyl acetate).b,cRepresents the signal-to-noise ratio (S/N) of diacetyl and acetoin, respectively. The absence ofS. thermophilusin the culture resulted in a lower accumulation of those compounds, whereas the absence ofL. cremorisled to their higher accumulation. The black horizontal line indicates the average value of the two compounds at milk prior to acidification. The box edges represent the interquartile range, the ends of the whiskers represent ± 1.5 × the interquartile range and central lines are the median values (as inf). Panels based onn= 3 biologically independent samples. Two-sidedttest were performed for each condition against the whole community (All). The symbols indicate the statistical significance results with ns:p> 0.05, *p< = 0.05 and **p< = 0.01.dSchematic compilation of the compounds that changed between the whole SLAB culture and whenL. cremoriswas left out (for detailed boxplots see Supplementary Fig. 8 & 10). The colour represents the removal conditions; orange indicates the removal ofL. cremoriswhile red represents the whole SLAB culture. The upwards arrow indicates the increase of the compounds relative to their compounds concentration in milk. The X symbol indicates the lack of production of the compounds in the respective condition.eSimplified metabolic Escher maps from citrate toα-ketoglutarate as well as to diacetyl through pyruvate and (S)-2-acetolactate. Metabolites and reactions are indicated by black and gray colour in the graph, respectively. Full coloured circles and open coloured circles indicate the high and low transcription per strain, respectively. The absence of circle indicates the lack of the corresponding orthologous group genes. Note that the transcriptional fluxes from the citrate-sodium symporter towards diacetyl are present in all members of theLactococcuscommunity. In addition, LC and LLm1 manifest higher transcription among theLactococcuscommunity on the genes related to acetolactate decarboxylase. Only LC strain within theLactococcuscommunity manifests transcriptional flux through diacetyl reductase and butanediol dehydrogenase as well as in reactions towardsα-ketoglutarate.fPredicted fluxes based on metabolic modeling across the different simulated media. 4 f–i, Supplementary Table 4 and Supplementary Note 2 ). The purine and pyrimidine biosynthesis pathways are deferentially expressed in a coordinated manner. Several genes in the pathways were up-regulated, in particular the genes associated with the reactions leading to uridine and guanine synthesis (Fig. 4 j and Supplementary Note 2 ). Both pathways are connected via L-glutamine synthetase. Expression patterns in amino acid metabolism show a mixed pattern of both up- and down- regulation (see Supplementary Note 2 ). Overall, the metatranscriptomics analysis further supports that S. thermophilus cross-feed Lactococcus community. Co-culture studies traditionally emphasized competitive interactions [25] , but recent evidence highlights the importance of cross-feeding cooperative interactions in community assembly [26] . Here, one hypothesis that could explain the identified cross-feeding interaction is that S. thermophilus has a higher proteolytic activity, thereby providing more peptides and amino acids (available nitrogen source) in the culture which Lactococcus takes advantage of [27] , [28] . When S. thermophilus is absent, there is a lower degree of nitrogen availability causing up-regulation of the nitrogen assimilation and nucleotide synthesis pathway in Lactococcus . A previous study conducted in a chemically-defined medium has also identified proteolysis and amino acid exchange as significant interactions between S. thermophilus and L. lactis [13] . Cheese flavour compounds are strongly influenced by the interactions within Lactococcus community To elucidate the role of interactions between the SLAB strains in the development of cheese flavour, we performed a targeted metabolomics analysis. Leaving out L. cremoris (LC) led to the strongest metabolic response followed by a weaker and different response when leaving out LLm1, S. thermophilus and the Lactococcus blend (see Supplementary Note 3 ). Surprisingly, leaving out LLm2 did not lead to a marked change in the metabolic profile of the acidified milk (Fig. 5 a). Six flavour compounds, namely heptanal, hexanal, 2-ethyl-furan, 2,3-pentanedione, diacetyl and acetoin, were either detected at significantly higher concentrations or only produced when this main L. cremoris strain was removed (Fig. 5 b, c and Supplementary Fig. 8 ). A graphical summary of the metabolome differences between the whole culture and the culture lacking LC is shown in Fig. 5 d. Many additional flavour compounds found were significantly altered by the strain removal strategy (Supplementary Fig. 9 – 10 and Supplementary Note 3 ), with the majority corresponding to byproducts of secondary metabolism with unknown microbial biosynthesis pathways or gene clusters. Yet, investigation of their patterns highlights the numerous ways these compounds may cross-feed within the SLAB culture. For example, 2,3-pentanedione could be cross-fed by S. thermophilus to LC, as it was found in milk only when S. thermophilus was present and in higher amounts when LC was absent (Supplementary Fig. 8 d). Alternatively, the observed pattern could be a result of substrate competition between the two strains. On the other hand, ethyl hexanoate, ethyl acetate and 2-methyl-3-thiolanone are likely produced by LC (Supplementary Fig. 10 a, b and d). Fig. 5: Cheese flavour compounds are strongly influenced by the interactions within Lactococcus community. The measured metabolome from the controlled milk experiments in response to strain removal conditions ( a–d ). a The PCA of key carbohydrades, acids and cheese flavour compounds. The strongest response was observed from the removal of L. cremoris , followed by a coordinated response of LLm1, LB and S. thermophilus . Removal of LLm2 does not affect the measured metabolome. The arrows represent the top 5 compounds responsible for the observed changes (2,3-pentanedione, hexanal, diacetyl, acetoin and ethyl acetate). b , c Represents the signal-to-noise ratio (S/N) of diacetyl and acetoin, respectively. The absence of S. thermophilus in the culture resulted in a lower accumulation of those compounds, whereas the absence of L. cremoris led to their higher accumulation. The black horizontal line indicates the average value of the two compounds at milk prior to acidification. The box edges represent the interquartile range, the ends of the whiskers represent ± 1.5 × the interquartile range and central lines are the median values (as in f ). Panels based on n = 3 biologically independent samples. Two-sided t test were performed for each condition against the whole community (All). The symbols indicate the statistical significance results with ns: p > 0.05, * p < = 0.05 and ** p < = 0.01. d Schematic compilation of the compounds that changed between the whole SLAB culture and when L. cremoris was left out (for detailed boxplots see Supplementary Fig. 8 & 10). The colour represents the removal conditions; orange indicates the removal of L. cremoris while red represents the whole SLAB culture. The upwards arrow indicates the increase of the compounds relative to their compounds concentration in milk. The X symbol indicates the lack of production of the compounds in the respective condition. e Simplified metabolic Escher maps from citrate to α -ketoglutarate as well as to diacetyl through pyruvate and (S)-2-acetolactate. Metabolites and reactions are indicated by black and gray colour in the graph, respectively. Full coloured circles and open coloured circles indicate the high and low transcription per strain, respectively. The absence of circle indicates the lack of the corresponding orthologous group genes. Note that the transcriptional fluxes from the citrate-sodium symporter towards diacetyl are present in all members of the Lactococcus community. In addition, LC and LLm1 manifest higher transcription among the Lactococcus community on the genes related to acetolactate decarboxylase. Only LC strain within the Lactococcus community manifests transcriptional flux through diacetyl reductase and butanediol dehydrogenase as well as in reactions towards α -ketoglutarate. f Predicted fluxes based on metabolic modeling across the different simulated media. Full size image C4 aroma compounds such as diacetyl and acetoin are known derivatives of citrate metabolism with characteristic contribution to buttery-like aroma. Although desirable in small quantities, e.g less than 0.05 mg. per 100 g of diacetyl content, higher amounts could lead to off-flavours [29] , [30] . Therefore, we investigated whether the increase in diacetyl and acetoin concentrations triggered by the removal of LC could be explained by the metatranscriptome profiles. Indeed, we found differential expression patterns in genes related to diacetyl and acetoin metabolism. We examined the gene expression levels in the metabolic route from citrate towards diacetyl and acetoin through pyruvate as well as an alternative route towards α -ketoglutarate. The citrate-sodium symporter that is present only on Lactococcus strains was highly expressed implying active uptake of the citrate available in milk by L. lactis . From citrate, Lactococcus strains showed expression of the genes associated with the pyruvate carboxylase and acetolactate synthase reactions, whereas only LC and LLm1 had the genes related to acetolactate decarboxylase expressed at high levels. On the other route towards α -ketoglutarate and further, genes associated with aconitate hydratase and isocitrate dehydrogenase are only expressed in LC and S. thermophilus (Fig. 5 e and Supplementary Figs. 11, 12 . Metabolic modeling simulations across the different medium conditions are largely corroborated by the metatranscriptomics results with the exception of three reactions involving acetoin. These are acetolactate decarboxylase (ACLDC), which does not carry a flux in the LC model, and 2,3-butanediol dehydrogenase (BTDD_RR) and diacetyl reductase (ACTD), which carry fluxes in LLm1 model but not in LC model (Fig. 5 e, f). Taken together, the presence of the main L. cremoris strain in the cultures results in the prevention of an undesirable increase in the levels of some key flavour compounds, including diacetyl and acetoin. This can be attributed to the degradation of diacetyl, e.g., through the action of some alcohol dehydrogenases from LC. Alternatively, LC might be competing with the other strains in the culture on citrate and subsequently converting it to other products than diacetyl and acetoin, such as ethyl-hexanoate, ethyl-acetate and 2-methyl-3-thiolanone, which normally happens in mixed culture fermentation following the rapid drop of redox potential in the beginning of fermentation [4] , [31] , [32] . This would result in the reduction of the overall amount of citrate available for diacetyl and acetoin formation. Microbial interactions as a mechanism in Cheddar cheese flavour formation Interactions in microbial communities are reported in a wide range of ecosystems [33] , [34] , [35] , [36] , [37] . While such interactions are widely reported also in food microbial communities [4] , [38] , [39] , [40] , [41] , [42] , very few studies have provided insights into the molecular agents that mediate the interactions. Uncovering interactions in situ is particularly challenging due to complexity of the communities involved as well as that of the medium such as milk. Here, we combined genomics, metatranscriptomics, metabolomics, and metabolic modeling to uncover key microbial interactions in Cheddar cheese-making. Notably, we used industrial strains and a full cycle of one-year long cheese ripening. In presence of S. thermophilus , we report a significant one-year long growth benefit to Lactococcus strain population, leading to a distinct final cheese metabolome profile. Based on these findings, we conclude that cross-feeding interactions within the SLAB culture substantially contribute to the formation of flavour in cheese. Our analysis indicated that S. thermophilus plays a crucial role by providing the necessary nitrogen source to the Lactococcus community. This provides an explanation about the observed growth benefit of the Lactococcus population and establishes a connection between the cross-feeding interactions and the development of cheese flavour. Additionally, we identified competitive metabolic interactions within the Lactococcus community. L. cremoris strain competes with L. lactis for the available citrate, resulting in accumulation of key metabolites such as diacetyl and acetoin in the final product. Such interactions take place within the first 5 hours of milk fermentation and strongly influences the final cheese flavour. Lastly, we have identified that the strains of Lactococcus affect the activity of S. thermophilus differently. While the presence of one L. lactis strain hardly influences the activity of S. thermophilus and the development of the final cheese flavour profile, the presence of a different L. lactis strain influences both significantly. Often in literature the attempts to study microbial interactions disregard the strain diversity. Yet, recent studies highlight the importance of strain interactions, claiming the major role of those in predicting eco-evolutionary dynamics [43] . Our results show how strain-specific metabolic interactions between microbes shape the biochemical profile of cheese, and provide targets towards the rational design and assembly of microbial communities with the aim of fine-tuning cheese flavour. More broadly, the study provides a blue-print to uncovering in situ interactions in complex food microbial ecosystems. Starter lactic acid bacteria culture A cheese making experiment was designed to investigate the effect of removing selected strains from a defined-strain SLAB culture. Wild-type strains were obtained from the Chr. Hansen Culture Collection and were originally isolated from dairy products or cultures. By applying this strain removal strategy, it becomes possible to gain insights into the individual role of the strain but also its interactions within the microbial community. The original defined-strain SLAB culture consisted of five different components: one component with single strain S. thermophilus , one component with a multi strain mixture of 21 Lactococcus strains belonging to both species of L. lactic and L. cremoris [44] , which were inoculated as a single component (hereafter, Lactococcus blend), two components with single strain L. lactis , and one component with single strain L. cremoris . The original defined-strain SLAB culture was composed of 25 strains and all bacterial and all strains applied are listed in Supplementary Table 1 . To apply the strain removal strategy four defined-strain SLAB cultures were designed. Condition ALL, corresponded to the original defined-strain SLAB composed of 25 strains packed under industrial conditions. Condition HP, corresponded to the original defined-strain SLAB composed of 25 strains packed under non-industrial condition by hand. Condition -LB, corresponded to the removal of the Lactococcus blend. Condition -ST, corresponded to the removal of the S. thermophilus strain. The amount added varied between the conditions to target the same acidification profile in the cheese vat while the cheeses making process was kept constant. The target was to obtain a pH of 5.35 at milling and a final moisture in non-fat solids of the cheeses at 54% ± 0.5% measured after 2 weeks of ripening. The designed defined-strain SLAB for conditions ALL, HP, and -LB were all dosed using 8.1 g of culture/100 L, whereas the designed defined-strain SLAB for condition -ST was dosed at a concentration of 17.3 g/100 L to compensate for missing contribution to acidification from S. thermophilus . The proportion of each component was adjusted based on the dosage recommended by the producer for the intended use expressed in terms of units of activity, as indicated on the component’s information sheet. The final compositions of each component within the SLAB cultures are provided in Supplementary Table 14 . Cheese making Cheeses were produced at the Application and Technology Center of Chr. Hansen A/S (Hørsholm, Denmark). The composition of the pasteurized cheese milk (organic milk, Naturmælk, Denmark) was measured using a Milkoscan™ (FOSS, Hillerød, Denmark), and the fat level was adjusted with pasteurized cream (organic cream 38% fat, Naturmælk, Denmark) to obtain a protein to fat ratio of 0.90. The cheese milk was heated to 32 °C and each cheese vat was filled with 150 kg. The milk was ripened for 40 min with the starter culture before the coagulant (CHY-MAX® Plus, Chr. Hansen A/S) was added. After 30 min of coagulation, the gel was cut into cubes 10 × 10 mm. The whey and the cheese grains were stirred for 10 min before heating to 38 °C over 40 min and the final scalding and stirring period was 45 min before whey drainage at pH 6.4–6.5. After 20 min, the cheese curd was cut into 12 blocks and rearranged in blocks 3 times during the next 75 min until pH 5.35 was obtained. The blocks where then milled, and the chips were dry salted (1.7–2.0% salt in dry matter) by manually adding and mixing the salt 2 times during 15 min. The salted chips were mixed every 5 min over a period of 30 min. Following molding, the chips were pressed at 2 bars for 15 min followed by 5 bars for 17 h. The cheeses were vacuum-packed and stored at 9 °C until sampling after 0.5, 3, 6, 9 and 12 months. The cheese gross composition (moisture, fat, protein and total solids) was estimated after 2 weeks of ripening by FoodScan™ (FOSS, Hillerød, Denmark). The NaCl content was estimated by analyzing the chloride concentration by automated potentiometric endpoint titration (DL50, Mettler-Toledo A/S, Glostrup, Denmark). pH was measured potentiometrically (PHC2002-8, Radiometer Analytical SAS, Lyon, France) in a paste prepared by mixing 10 g of grated cheese with 10 ml of deionized water with a wooden spatula. All analyses were carried out in duplicate. In summary, for the one year-long ripening cheese making experiment we inoculated three variations of the SLAB cultures into four milk tanks. Two milk tanks were inculcated with the complete set of strains, one used as the control and the other to test a different approach of culture inoculations (All and All HP, respectively). The two other variations of the culture were prepared using the ‘strain removal strategy’ with the aim of testing the effect of L. lactis blend (All-LB) and of the single S. thermophilus (All-ST) during cheese-making. Following the acidification phase, we sampled the resulting cheddar cheeses in 5 time points over the one year period. We followed two batch experiments started on two consecutive days. Microbial community dynamics Grated cheese (5.0 g) was mixed with 45.0 g of autoclaved 2% sodium citrate buffer, pH 7.5, 46 °C. The mixture was homogenized in a Stomacher® blender for 4 min at medium setting to dissolve the cheese and suspend the bacteria present. Sequential 10-fold dilutions were prepared as required in 0.1% peptone/0.15M NaCl in water, pH 7.0. The total population of Mesophilic cocci ( Lactococcus ) was determined on pour plated M17 Agar (Difco, USA) after aerobic incubation for 5 days at 30 °C. The total population of Thermophilic cocci (ST) was determined on pour plated M17 Agar after aerobic incubation for 3 days at 37 °C. The total population of non-SLAB was determined on overlaid Rogosa Agar (Sigma Aldrich, USA) after incubation for 7 days at 37 °C. The microbial analysis was carried out in duplicate at each sampling point. Carbohydrates and organic acids in cheese The content of lactose, glucose, galactose, lactate, citrate and acetate were quantified using a Dionex ICS-3000 RFIC-EG™ dual system equipped with an amperometric detector (Dionex, Sunnyvale, CA, USA). The separation was performed using an anion-exchange column (CarboPac® PA20, 3 × 150 mm, 6.5 μm) and an ion-exclusion column (IonPac® ICE-AS6, 9 × 250 mm, 8 μm). Grated cheese (3.0 g) was mixed with 15 ml 83 mM PCA containing  mM Na-EDTA, 30 mM arabinose and 48 mM 2-hydroxyisobutyric acid (internal standards) and rotated for 30 min at room temperature. This extract was subsequent centrifuged (5000 × g, 30 min, 4 °C) and the supernatant was filtered (0.45 μm). The supernatant was diluted (600-fold) before analysis. For analysis of carbohydrates 25 μL was injected and the separation was performed at 26 °C with a flow rate of 1.3 mL/min increasing the KOH concentration as follow: 1 mM KOH for 5 min, from 1 mM to 20 mM KOH over 0.5 min, then kept at 20 mM KOH for 6.6 min min before re-equilibration to 1 mM KOH over 5 min. For analysis of organic acids 50 μL was injected and the separation was performed at 30 °C with a flow rate of 1 mL/min using 0.4 mM heptfluorobutyric acid in 5% acetonitrile as eluent. The analysis was performed in duplicate at each sampling point. Proteolysis in cheese Grated cheese (2.0 g) was mixed with 18 ml distilled water and blended for 2 min at 25,000 rpm (Ultra-Turrax model T25). This suspension was used for determination of total nitrogen (TN), Non-Casein nitrogen (NCN), and non-protein nitrogen (NPN) using the fractionation procedure described in standard NF ISO 27871 (ISO, 2011). The nitrogen content for each fraction was determined using the Kjeldahl method as described in standard NF EN ISO 8968-1 (ISO, 2014). The level of primary proteolysis (NCN) and secondary proteolysis (NPN) were expressed as the percentage of TN found in the cheese. The analysis was performed in duplicate at each sampling point. Peptides in cheese The peptide profile was analyzed by liquid chromatography-mass spectrometry (LC-MS/MS). Grated cheese (3.0 g) was mixed with 15 ml urea solution (8 M urea, 0.01 M HCL, 0.1% DTT) and rotated for 30 min at room temperature. This extract was subsequent centrifuged (5000 × g, 20 min, 4 °C). 1 ml of the supernatant was transferred to an Eppendorf tube and centrifuged (12,000 × g, 5 min, 4 °C). The supernatant was transferred to vial ready for analysis. Separation was performed using an Agilent 1290 Infinity UHPLC (Agilent, Santa Clara, USA). Injection volume was 3 μL and the peptides were separated using a reversed-phase column (Waters Acquity CSH C18 peptide column (1.7 um, 2.1 × 150 mm). Binary linear gradient elution at 50 °C was applied by mixing MilliQ water (0.1% formic acid) (A) with acetonitrile (0.1% formic acid)(B). The gradient used was as follows: 0–0.36 min 96% A, 70% A at 8 min, 54% A at 14 min, 20% A at 16 min, holding 20% A until 16.5 min, increasing to 96% A at 16.6 min and holding until 21 min. The flow rate was 0.3 mL/min. Detection was performed using an Agilent 6540A quadrupole time-of-flight (QTOF) mass spectrometer (Agilent, Santa Clara, USA). Mass spectra were acquired using electrospray ionization in positive mode in the mass range m/z 100–3000. MS/MS analysis was performed using collision induced fragmentation using data-dependent acquisition. For each MS full scan, the two highest intensity ions were selected for fragmentation. The mass of the peptides was annotated using MassHunter Bioconfirm (ver. B.10.0, Agilent Technologies) and quantification by MassHunter Qualitative analysis (ver. B.09.00, Agilent Technologies). The peptide masses were assigned to particular sequences of dairy proteins using Peak Studios (Bioinformatics Solutions Inc.). The data base search was performed using a 50 ppm threshold on mass accuracy and a 0.3 Da threshold on the fragment ions. The digestion enzyme was set to none leading to an unspecified digestion pattern. The analysis was performed in duplicate at each sampling point. Free amino acids in cheese The content of free amino acids (not arginine, but including the breakdown product ornithine), γ -amino butyric acid (GABA), and biogenic amines (phenylethylamine, putrescine, putrescine, cadaverine, histamine, tyramine, spermidine) were quantified using gas chromatography-mass spectrometry (GC-MS) (7890A & 5975C, Agilent Technologies). Grated cheese (3.0 g) was mixed with 15.0 ml milli-Q-water and rotated for 30 min at room temperature and subsequent centrifuged (5000 × g, 30 min, 4 °C) and the supernatant was filtered (0.45 μm). For each sample, 25 μL were mixed with 225 μL milli-Q-water, 50 μL 1.72% norvaline as internal standard, 200 μL of methanol/pyridine 32/8% (v/v). Subsequently, 25 μL methyl chloroformate was added and mixed using a whirlmixer at 3000 rpm for 5 s. Then, 500 μL 1% mff/choloroformate was added and the sample mixed using a whirlmixer at 3000 rpm for 5 s. For the analysis 2 μL was injected unto a DB-XLB 15 m × 0.25 mm x 0.25 μm column (Agilent Technologies) using helium as carrier gas, flow of 1.26 mL/min and an own program of 110 °C (0 min) with a gradient of 20 °C/min until 320 °C (0 min). The analysis was performed in duplicate at each sampling point. Volatile compounds in cheese Volatile compounds were analyzed using Solid Phase Micro Extraction (SPME) and GC-MS (7890B & 5977A, Agilent Technologies) equipped with a SPME autosampler (Gerstel). A plug of cheese (3.0 g) was transferred using a syringe to a 20 ml vial and 100 μL internal standard was added before closing the vial with a cap. The internal standard consisted of a 10 ppm solution of ethanol-d6, dimethyl-d6-disulfide, 2-methyl-3-heptanone and pyrazine-d4 solubilized in 1-methyl-2pyrrolidone. The vial was heated at 60 °C for 10 min and volatiles were adsorbed to the SPME fiber (DVB/Car/PDMS Gray, 2 cm, Supelco) using an extraction time of 20 min. The fiber was transferred to the GS-inlet and kept at −50 °C for 2 min and then the temperature was increased at 16 °C/s to 150 ∘ C and then 12 °C/s to 300 °C, leading to desorption of the volatiles. Volatiles were then separated on a DB-5, 30 m × 0.25 mm × 1 μm column (Agilent Technologies) using helium as a carrier gas 0.085 ml/min at 325 °C. The mass spectra of the volatile components were collected by running MS scans within the mass range of m/z 29–209. The volatiles were identified by comparison of mass spectra using a compound specific quantifier ion and 2 qualifier ions within a given retention index window. This was done using MassHunter (Version B.07.02.1938, Agilent Technologies). Results were given as signal-to-noise (S/N) which was calculated as peak height divided by baseline noise. Cheeses from the sampling points 3, 6, 9 and 12 months were analyzed in duplicate. The measurements for the second week are missing for volatile compounds, as they are expected to be very limited. Finally, the metabolic profile of the cheeses was quantified by measuring 30, 3, 28 and 248 features belonging to the classes of acids, sugars, flavour-related organic compounds and peptides, respectively. Genome sequencing and assembly Genomic DNA for de novo short read whole-genome shotgun sequencing was extracted from 1 mL of overnight culture (M17 Broth (Difco) supplemented with glucose) of each of the strains (at OD600 = 1) with DNeasy Blood and Tissue kit on QiaCube system (Qiagen, Germany) following the manufacturer’s protocol. Prior to extraction, cell pellets were washed twice in TES buffer (50 mM TRIS pH 8.0, 1 mM EDTA pH 8.5, 20% sucrose) and then resuspended in 180 uL of pre-lysis TET buffer (20 mM TRIS-Cl pH 8.0, 2 mM EDTA pH 8.5, 1,2% Triton X-100, 20 mg/mL lysozyme, 2 μL of 25 U/μL mutanolysin, 4 μl of 100 mg/mL RNase A). Genomic libraries were prepared using KAPA LTP Library Preparation Kit KK8230 (Roche, Switzerland) on a Biomek 4000 Liquid Handler (Beckman Colter, USA). A portion of 500 ng of genomic DNA diluted in EB buffer (Tris-Cl, pH 8.0) was mechanically fragmented on Bioruptor® Standard (Diagenode, USA) with 12 sonication cycles (30 s ON/OFF) to obtain an average fragment size of 300 bp (CV%: 1.5). Fragmented DNA was processed following the KK8230 kit manufacture’s protocol. Following the adapter ligation step, adapter-modified DNA fragments were enriched by 8-cycle PCR. AMPure XP (Beckman Colter) paramagnetic beads were used for clean-ups to purify fragments at average size between 450 and 550 bp. Concentration of gDNA and double stranded DNA libraries were measured by Qubit® Fluorimeter using Qubit dsDNA Broad range and Qubit 1 × dsDNA HS assays (Thermo Fisher Scientific, USA), respectively. Average dsDNA library size distribution was determined using an Agilent HS NGS Fragment (1–6000 bp) kit on an Agilent Fragment Analyzer (Agilent Technologies, USA). Libraries were normalized and pooled in NPB solution (10 mM Tris-Cl, pH 8.0, 0.05% Tween 20) to the final concentration of 10 nM. Following denaturation in 0.2 N NaOH, 10 pM of pooled libraries in 600 μL ice-cold HT1 buffer were loaded onto the flow cell provided in the MiSeq Reagent kit v3 (600 cycles) and sequenced on a MiSeq platform (Illumina Inc., San Diego, USA) with a paired-end protocol and read lengths of 301 nucleotides. All processing of the short reads was done in either CLC Genomics Workbench versions 9.5.3, 9.5.4 or 10.1.1. The short reads were mapped with default parameters to the reference sequence of the phage Phi × 174 using the tool “Map reads to reference”. Unmapped reads from the mapping were trimmed for quality using the PHRED score 23 as the threshold and with the non-default parameter of discarding reads that were less than 50 base pairs long using the tool “Trim Sequences”. The trimmed reads were de novo assembled with default parameters except for the minimum contig length was set to 600 base pairs using the tool “De Novo Assembly”. Afterwards, a decontamination step was performed where contigs with low depth of coverage were removed using a custom plugin written by Qiagen. The decontamination step first removes all contigs where the depth of coverage is below 15X and afterwards removes all contigs where the depth of coverage is below 25% of the median depth of coverage for the entire genome assembly. Gene calling of the filtered contigs was done with Prodigal version 2.6.2 using the default parameters. Finally, the genome assemblies with annotated genes were functionally annotated with BLAST against a local annotation database using a custom plugin written by Qiagen. Comparative genomics and phylogenomics A L. lactis and L. cremoris pan-genome was created without strain LC-LB16 which was found to have 6 times more singletons than all the other strains. The number of core, accessory, and unique (singletons) genes in the pan-genome is 1247, 3308, and 2323, respectively. The OGs from this pan-genome were used in the comparative genomics and differential metatranscriptome analyses as well as in the creation of a pan-metabolic network of L. lactis and L. cremoris for microbial community modeling. We identified all k-mers of length up to 31 bps ( k = 31) in the genomes of all the strains and unique k-mers in each strain were filtered. For the set of unique k-mers we mapped the metatranscriptomic reads to get their abundance and kept only those above seven counts. Normalization of the number of counts per strain performed based on the number of unique k-mers identified in each of the strains. From the total pool of 54667 genes 15.8% was removed as the cluster above 96 cd-hit identity was mixed among the three taxa. still 84.2% consider a significant number to look at L. cremoris and L. lactis differences. For the phylogenetic analysis 22 genomes from the SLAB culture were used alongside 107 complete genomes of L. lactis and L. cremoris , which were retrieved from NCBI results in total to 129 genomes. CD-HIT (v4.8) on 80% amino acid identity thresholds along with a custom-made R script were used to identify a set of 464 monocore marker gene sets [45] , [46] . The trees were constructed using PhyloPhlAn v3.0 [47] using the PhyloPhlAn parameters “–accurate” and “–diversity low”, which translate to the usage of a pfasum60 substitution matrix. In addition, multiple sequencing alignments (msa) were performed with muscle (v3.8.1551) and trimming was performed by removing columns with at least one nucleotide appearing above a threshold of 0.99. The final maximum likelihood tree was constructed on the concatenated DNA msa using raxmlHPC (v8.2.12), 100 bootstrap and GTRGAMMAI model [48] , [49] . Generation and simulation of genome-scale metabolic models The metaGEM workflow’s prokaryotic GEM reconstruction and simulation module was used for metabolic modeling [50] . Genome-scale metabolic models were generated for S. thermophilus , Lactococcus LLm1, LLm2, and LC using CarveMe v1.4.1 [51] based on the protein sequences of assembled genomes. First, Prodigal v2.6.3 [52] was used to generate open-reading-frame annotated protein sequence files from the corresponding DNA fasta files. Additionally, milk media from a recent kefir publication was used for gap-filling during model generation [42] . More specifically, we formulated four biologically relevant variations of the milk composition, including aerobic rich milk, anaerobic rich milk, aerobic depleted milk, and anaerobic depleted milk. The former two media represent the initial composition of milk, while the latter two media represent milk after it has been depleted by fermentation. A version of each of the four species was generated by gap-filling on each of the four milk media variations, as well as without gap-filling, resulting in a total of 20 models. All models were generated using the default CarveMe universal bacterial model template. Note that although gram positive bacteria are generally not modeled with a periplasmic compartment due to its smaller size relative to gram positive bacteria, all models generated with the automated CarveMe tool contain such a compartment. Individual model simulations were carried out for all models on each of the four media variations using the reframed v1.2.1 and cobrapy v.0.20.0 metabolic modeling packages [53] . Community simulation of genome-scale metabolic models was also carried out in the different media variations, using SMETANA v1.2.0 [22] . All associated data, including code used for generating and plotting results, is available on GitHub. Inoculations in milk All milk fermentations were carried out in organic low fat (1.5%) milk from the organic dairy NATURMÆLK, Tinglev, Denmark, which consists of skim milk powder at a level of dry matter of 9.5% (w/v) reconstituted in distilled water and pasteurized at 99 °C for 30 min, followed by cooling to 30 °C [54] . Starting material for all inoculations were concentrated F-DVS® (Direct Vat Set) strains and cultures for direct inoculation into. All cultures were inoculated 0,02% with F-DVS material by firstly transferring 2.0 g F-DVS material to 200 ml cold milk. After mixing, 4 ml were transferred to 200 ml pre-warmed milk (32 °C) for the final fermentation. The percentages of the different strains and cultures for the 6 different culture blends is given in Supplementary Table 15 . Milk acidifications and sampling For the SLAB cultures, after inoculation into bottles with milk placed at 32 °C in a waterbath, pH measurement was started and acidification was followed using a CINAC system [55] . After 59 min, the temperature was raised to 38 °C and at 183 min, the temperature was reduced to the final temperature, 35 °C, for 20 h. The six different culture blends were each run in triplicate. After around 5 h of acidification during the exponential growth phase when reaching pH 5, 1 g fermented milk from each fermentation and 1 g unfermented milk were sampled and added 200 μl 4 N H2SO4 to prepare for analysis for organic acids, Carbohydrates and Volatiles. In addition 1 g was sampled for mRNA extraction. Temperature stress of individual Lactococcus strains was assessed by following the acidification of the same milk on four temperatures (30 °C, 37 °C, 40 °C and 43 °C) by continuous monitoring the milk’s pH levels. Carbohydrates, acids and volatiles in milk For the preparation of fermented milk samples used for carbohydrate and small organic acid analysis, 1 g or 1 mL of sample was quenched with 200 μL 4N sulfuric acid (H2SO4) in a 7 mL glass tube, mixed and stored at −20 °C until analysis. The analytes for carbohydrate analysis were extracted from the sample and proteins get deproteinated and precipitated by treatment with an aqueous perchloric acid (PCA) solution. The samples get further diluted to fit into the dynamic range of the quantification. Arabinose is added as an internal standard. The diluted samples are analyzed on a Dionex ICS-3000 system (Thermo Fischer Scientific, Waltham (MA), USA) using an analytical anion-exchange column and a pulsed amperometric detector. For quantification a one-point calibration curve is used. Concentrations are calculated based on the chromatographic peak heights after normalizing to the internal standard (arabinose). The analytes for analysis of small organic acids were extracted from the sample and proteins get deproteinated and precipitated adding an aqueous PCA solution. The samples get further diluted to fit into the dynamic range of the quantification. Adipic acid is added as an internal standard. The diluted samples are analyzed on a Dionex ICS-3000 or ICS-5000 system (Thermo Fischer Scientific, Waltham, MA, USA) using an analytical ion exclusion column and a suppressed conductivity detector. For quantification, an 8-point calibration curve is used. Concentrations are calculated based on the chromatographic peak heights after normalizing to the internal standard (adipic acid). For the preparation of the volatile organic compounds (VOC’s) samples, 1 g or 1 mL of each sample was transferred to a head space vial (20 mL) with 200 μL of 4N H2SO4 and sealed with teflon-lined aluminum caps. The samples were then identified using a static head space sampler connected to a Gas Chromatograph with Flame Ionization Detector (GC-FID) (Perkin Elmer, MA, USA) and equipped with a HP-FFAP column. The identification of VOC’s was based on retention time in comparison with that of standards. The injector and detector were maintained at 180 °C and 220 °C, respectively. The oven was initially heated to 60 °C and held for 2 min, then increased to 230 °C and held for 0.5 min. The calculation of the concentration of each compound in each sample was based on the peak height divided by the response factor. The response factor is established suing standard solutions by the quotient of the peak height divided by the known sample concentration. All of the chemicals and analytes used for the standard solutions were provided by Sigma-Aldrich, Munich, Germany. Overall with these approaches, we measured a total of 43 metabolites comprising five carbohydrates, eight organic acids and 30 important flavour compounds. RNA extraction, sequencing and analysis Total RNA was extracted using the RNeasy Mini kit (Qiagen 74104) and rRNA was depleted with the NEBNext rRNA Depletion Kit (Bacteria). The sequencing library was then prepared using the NEBNext Ultra II Directional RNA Library Prep Kit for Illumina and the libraries were sequenced by EMBL Genomic C-ore Facility using the Illumina NextSeq 500 system, read length 150 bp. The RNA-reads are preprocessed and filtered based on minimum quality and length using the NGLess pipeline and substrim. Given a read it finds the longest substring, such that all bases are of at least the given quality. The parameters minimum quality and minimum length were set to 25 and 100, respectively. The filtered reads are mapped to the genomes of all strains present in the Culture using bbmap (v38.75)—if one read has multiple hits, a random distribution is used (selecting one top-scoring site randomly). The total number of reads ranges from 4,855,868 to 18,812,096 in samples 4B and 1B, respectively, and the percentage of mapped reads is in the range of 93–95% (Supplementary Table 16 ) [56] . htseq-count (v0.11.2) was used to count the number of reads per gene [57] . The resulting counts were grouped per orthology group (custom python script) based on a previously created pan-genome created for the pan-metabolic network. Normalization was performed and differential gene expression with DESeq2 (v1.26.0) and SARTools (v1.7.2) in R [58] , [59] . For the differential gene expression analysis, Wald significance tests were performed with BH p -value adjustments [60] to take into account multiple testing, and the level of controlled false positive rate was set to 0.01. Further differentially expressed genes, Lactococcus pan-metabolic network information and KEGG pathways were based on custom analysis [35] , [61] . The data was normalized using DESeq2 to correct systematic technical biases and make it possible to compare read counts across samples. The median scaling factor for each sample was used. This is done for the data containing all genes. RegPrecise database was used for validation of key functional regulation [62] . General statistical and computational analysis We used R-packages Boruta (v8.0.0), uwot (v0.1.14), apcluster (v1.4.10), ggplot2 (v3.4.2), ggrepel (v0.9.3), ggfortify (v0.4.16), ggridges (v0.5.4), ggbiplot (v0.55), ggpubr (v0.6.0), ggalluvial (v0.12.5), scales (v1.2.1), tidyverse (v2.0.0), dplyr (v1.1.2), plyr (v1.8.8), reshape2 (v1.4.4), cowplot (v1.1.1), patchwork (v1.1.2), rstatix (v0.7.2), viridis (v0.6.3), grid (v4.2.2), Biostrings (v2.64.1) and readxl (1.4.2) for downstream analysis including, data parsing and visualization, clustering, dimensionality reduction and importance feature ranking analysis [46] , [63] , [64] , [65] , [66] , [67] , [68] , [69] , [70] , [71] , [72] , [73] , [74] , [75] , [76] , [77] , [78] , [79] , [80] , [81] , [82] , [83] . Specifically, Boruta algorithm is a wrapper around Random Forest [84] that performs randomization tests. It is used to identify discriminative metabolites in cheese ripening experiment. Features with confidence of importance above 0.99 (the default value in Boruta) were treated as informative. Also the maximal number of importance source runs was increased to 10,000. In this study, statistical analysis of variance (ANOVA) and pairwise comparisons between two groups using either the Wilcoxon rank-sum test (wilcox.test) or the Student’s t test ( t test) were conducted. The resulting p -values were reported in the figures. Temperature stress of Lactococcus strains was represented as a proxy based on the Pearson correlation coefficient (PCC) between the acidification curves of mono-cultures at 30 °C compared to mono-cultures at 37 °C, 40 °C and 43 °C. Metabolic networks were visualized using Escher web-tool (v1.5.0) [85] . Schematic representations and figures were created and polished, respectively, in Inkscape. Reporting summary Further information on research design is available in the Nature Portfolio Reporting Summary linked to this article.